Encapsulation of sulfur with thin-layered nickel-based hydroxides for long-cyclic lithium–sulfur cells Elemental sulfur cathodes for lithium/sulfur cells are still in the stage of intensive research due to their unsatisfactory capacity retention and cyclability. The undesired capacity degradation upon cycling originates from gradual diffusion of lithium polysulfides out of the cathode region. To prevent losses of certain intermediate soluble species and extend lifespan of cells, the effective encapsulation of sulfur plays a critical role. Here we report an applicable way, by using thin-layered nickel-based hydroxide as a feasible and effective encapsulation material. In addition to being a durable physical barrier, such hydroxide thin films can irreversibly react with lithium to generate protective layers that combine good ionic permeability and abundant functional polar/hydrophilic groups, leading to drastic improvements in cell behaviours (almost 100% coulombic efficiency and negligible capacity decay within total 500 cycles). Our present encapsulation strategy and understanding of hydroxide working mechanisms may advance progress on the development of lithium/sulfur cells for practical use. Lithium/sulfur (Li/S) cells are promising energy storage devices to power electric vehicles for long-distance driving (>300 miles per charge) due to their upper theoretical energy density and lower price in comparison with currently used Li-ion cells [1] , [2] , [3] . According to charge/discharge voltage profiles or electrolytes applied in Li/S cell systems, the cathode materials can be generally categorized into two types: (1) the elemental sulfur (aggregated cyclo-octasulfur S 8 ) and (2) a series of sulfur-derived composites [4] . Elemental S 8 owns overwhelming advantages over the synthetic thionic composites. On one hand, it is environmentally benign and abundant in nature, hence readily available and fairly cheap in markets; on the other hand, when coupled with Li metal anode, it operates at a safer voltage of ∼ 2.15 V (versus Li/Li + ) compared with conventional Li-insertion compounds ( ∼ 3–4.5 V versus Li/Li + ), and offers a higher energy density than thionic counterparts [4] , [5] , [6] , [7] . The S 8 can exhibit a total theoretical capacity of 1,672 mAh g −1 when undergoing an overall redox reaction of S 8 +16Li + +16e − ↔8Li 2 S (ref. 8 ). The corresponding energy density reaches as high as ∼ 2,567 Wh kg −1 , more than sixfold that of commercial LiCoO 2 /C cells ( ∼ 387 Wh kg −1 ) [9] . The development of Li/S cells based on pure S 8 cathode, however, is impeded by several challenges unfortunately. Primarily, both S 8 and the discharged end products Li 2 S 2 /Li 2 S are insulators [10] . Particularly noteworthy is that, Li 2 S is an extremely poor electrically/ionically conducting material with electrical conductivity of ∼ 10 −30 S cm −1 and Li + diffusivity of ∼ 10 −15 cm 2 s −1 , which inevitably poses inferior cell kinetics on charge transfer and low utilization efficiency of S 8 (ref. 3 ). Next is the undesired self-discharge issue in Li/S cells. Unlike LiCoO 2 /C cells with stable passivation layers covering on electrode interfacial surfaces, in Li/S cell system, the S 8 cathode exposed in electrolyte under a fully charged state tends to react with Li + gradually, convert to polysulfide species and dissolve into the electrolyte, which eventually results in a static energy decrease in cell capacity [11] . Last but the foremost, along repeated charge/discharge procedures, the unavoidable dissolution and loss of intermediate polysulfides (Li 2 S n , n =3–8), together with their notable ‘shuttle effects’ between the anode and cathode, will inevitably lead to the formidable issues of severe capacity decay, low coulombic efficiency and limited cyclic life [12] , [13] , [14] . The long-lasting and stable cyclic behaviour is undoubtedly the fundamental prerequisite for future commercialization of Li/S cells. To prolong the cyclic lifetime, a worldwide-recognized approach is to wrap the active S 8 with an effective physical barrier so as to solidly confine the soluble intermediate polysulfides in the cathode region [3] , [15] , [16] , [17] , [18] , [19] , [20] , [21] , [22] , [23] , [24] , [25] , [26] , [27] . Several S 8 encapsulation avenues have been presented to date, normally by the use of carbon materials (typically like two-dimensional graphene), conductive polymers or diverse inorganic coating layers [15] , [16] , [17] , [18] , [19] , [20] , [21] , [22] , [23] , [24] , [25] , [26] , [27] . Though using intrinsically mesoporous carbons is taken for granted as an ideal strategy to restrict polysulfide molecules in cathode matrices [15] , [16] , [17] , [18] , [19] , actually weak interactions between non-polar carbon materials and Li 2 S n reduce the ability to bind and entrap these soluble polar species [20] . As a consequence, only use of carbon materials can benefit the cell kinetics/reversibility and alleviate the capacity fading but still fail to resolve the short cyclic problem. Though soft conductive polymers or organic frameworks are also conceived as preferred and competitive inhibitors to hinder the polysulfides shuttling, their behaviours on elongating the cell lifetime are yet far from perfect [21] , [22] , [23] , [24] . By contrast, encapsulations realized via inorganic species (for example, S 8 –TiO 2 yolk–shell nanoarchitectures) hold great potential to build long-term cyclic Li/S cells [25] , [26] , [27] . Nevertheless, such state-of-the-art core–shell nanohybrids yet show little promise in broad commercial use owing to limitations such as low tap density and high surface areas of nanomaterials [28] , excess interparticle boundaries contained in electrode systems [29] and so on. Therefore, to overcome the major cyclic constraint and bring Li/S cells a step closer to commercialization, seeking for reliable ‘armors’ fit for S 8 cathode and an efficient encapsulating strategy applicable to bulks ( ∼ 20 μm scale) for higher volumetric energy is urgently pursued. Herein, we demonstrate the feasibility of adopting semiconducting nickel nitrate hydroxide (Ni 3 (NO 3 ) 2 (OH) 4 , denoted as NNH), one type of thin-layered α-Ni(OH) 2 often applied in nickel–metal hydride cells and supercapacitors, as a novel and effective encapsulation material for S 8 cathode. More than a durable physical shell, NNH is capable to irreversibly react with Li + in initial tens of cycles, turning into reliable (Li, Ni)-mixed hydroxide compounds with a combination of good Li + permeability/accessibility and copious functional polar/hydrophilic groups (for example, hydrophilic groups, surface hydroxyl groups and so on) existing in cathode systems [12] , [27] . In this work, we choose the simple hybrid of S 8 @carbon black (S 8 @CB; with a central dimension of ∼ 20 μm), as a paradigm to investigate the electrochemical functions of NNH. By using such a smart core–shell S 8 @CB@NNH hybrid as the cathode, we eventually achieve drastic improvements in capacity retention (almost ∼ 500% capacity rise when compared with the case of bare S 8 @CB) and long-term cyclic stability (negligible capacity decay within total 500 cycles). Our present work may open up a feasible and effective concept of using thin-layered transition metal hydroxides as a promising class of encapsulation materials to build better Li/S cells. Synthesis and characterization The entire fabrication of core–shell S 8 @CB@NNH bulky hybrids was schematically shown in Fig. 1a (see Methods section for details; basic characterizations on NNH are involved in Supplementary Fig. 1 ). In brief, the preparation of S 8 @CB particles was achieved by impregnation of molten S 8 into CB matrices. The choice of CB powder, which has been long commercialized in cell technologies, as the S 8 carrier is due to its large surface-to-volume ratios, excellent electrically conducting properties and far lower cost than other counterparts like advanced mesoporous carbons, graphene and carbon nanotubes and so on. Another notable reason is that there are numerous nanosized cavities ( Fig. 1b,c ) distributed in between CB nanoparticles, as reflected by the pore-size distribution plot ( Supplementary Fig. 2 ). These interspaces (randomly distributed in a wide range of ∼ 1–50 nm) can not only supply abundant ‘reservoir’ places to accommodate S 8 but also help to downsize the S 8 bulks into nanoparticles for preferable cell kinetics. 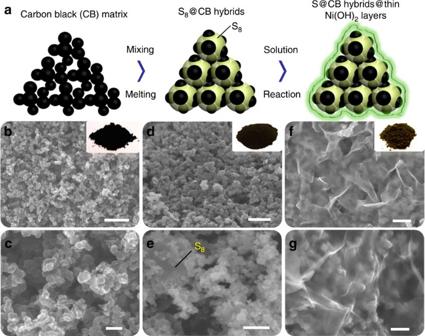Figure 1: Schematic and s.e.m. images showing the fabrication of S8@CB@NNH hybrids. (a) A general schematic for the entire fabrication procedures. Basic s.e.m. observations towards (b,c) CB powders, (d,e) S8@CB intermediates and (f,g) S8@CB@NNH hybrids. The inset pictures correspond to their optical images, respectively. Scale bars, 200 nm (b,d), 50 nm (c,g) and 100 nm (e,f). Figure 1d,e shows typical scanning electron microscopy (SEM) observations on S 8 @CB powders. During the melting treatment, the S 8 powders have definitely fused into a liquid state, penetrated/embedded into certain cavities and merged together with CB-conducting agents. The size for entire bulks is centred at ∼ 20 μm ( Supplementary Fig. 3 ), while the diameter of individual S 8 @CB subunit lies in a range of ∼ 20–100 nm. The following procedure was undertaken at a low temperature of 95 °C in an aqueous solution where the S 8 @CB hybrids are uniformly packaged by NNH. The reaction of Ni salts with ammonium (NH 4 OH) yielded from the progressive hydrolysis of hexamethylenetetramine (C 6 H 12 N 4 +10H 2 O→6HCHO+4NH 4 OH) guarantees an intact encapsulation of NNH layers on each S 8 @CB particle. Fresh S 8 @CB@NNH products are then washed by centrifugation and dried at 60 °C in an electronic oven. S.e.m. observations ( Fig. 1f,g ) reveal that the as-formed S 8 @CB@NNH hybrids possess a well-defined core–shell configuration; all of the nanosized S 8 @CB subunits have been intimately packaged within the layered film structures. Also, the stepwise evolutions of S 8 @CB@NNH are further confirmed in parallel using energy dispersive X-ray spectroscopy (EDX) to monitor the entire fabrication flow (see details in Supplementary Fig. 4 ). Figure 1: Schematic and s.e.m. images showing the fabrication of S 8 @CB@NNH hybrids. ( a ) A general schematic for the entire fabrication procedures. Basic s.e.m. observations towards ( b , c ) CB powders, ( d , e ) S 8 @CB intermediates and ( f , g ) S 8 @CB@NNH hybrids. The inset pictures correspond to their optical images, respectively. Scale bars, 200 nm ( b , d ), 50 nm ( c , g ) and 100 nm ( e , f ). Full size image A special focus is then put on the ultimate products of S 8 @CB@NNH. 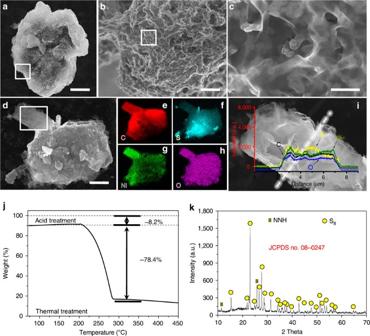Figure 2: Characterizations of the S8@CB@NNH bulky hybrids. (a–d) S.e.m. images of S8@CB@NNH hybrids. (e–h) EDX elemental mapping records towards one typical S8@CB@NNH bulky sample, and (i) a line-scan analysis on a selected section of this hybrid product. (j) A plot recording weight losses of S8@CB@NNH products during an acid immersion treatment combined with a TG measurement. (k) XRD pattern of synthesized S8@CB@NNH powders. Scale bars, 10 μm (a,d), 1 μm (b) and 100 nm (c). Figure 2a–d shows their basic s.e.m. observations. The large-area SEM detection ( Fig. 2a ) illustrates that the self-assembled S 8 @CB@NNH product owns a bulky structural feature ( ∼ 20 μm upward in width) and an interesting heart-shaped geometric profile. No naked areas are observed on bulky S 8 @CB@NNH hybrids, ascertaining our success in perfectly packaging S 8 @CB into NNH shells. Close-up s.e.m. images ( Fig. 2b,c ) furthermore uncover their detailed structural information. Definitely, every S 8 @CB nanoparticle unit has been overall and closely wrapped with NNH ‘armors’, as also confirmed by transmission electron microscope (TEM) image in Supplementary Fig. 5 . Note that our used encapsulating material is supple enough to conform well to arbitrary body shapes of introduced precursors, enabling a tight and intact encapsulation of involved S 8 @CB powders. Moreover, the NNH films are extremely thin (the thickness for one NNH layer is only ∼ 7 nm, as evidenced by pioneering works) [30] , [31] ; TEM and s.e.m. observations ( Supplementary Figs 1e,f and 6 ) further reveal the distribution of pore defects on NNH surface. Such a thin-film characteristic, together with intrinsic porosity properties (for example, micropores/mesopores on NNH or in between these overlaid structures) may allow Li + to move readily across the outer protective layers, pledging the expedite ionic access/permeation to inner places of entire cathode. Figure 2e–h displays the EDX elemental mapping records towards one bulky S 8 @CB@NNH product (see its SEM morphology in Fig. 2d ). The mapping images visually declare a homogeneous dispersion of C, S, Ni and O atoms in this hybrid. In addition, we purposely carry out a line-scan analysis on a selected section of S 8 @CB@NNH ( Fig. 2i ). Though there is a visible thick layer of NNH covering this region, the involved S element still takes up the largest proportion (rather than Ni or O element) and stays evenly distributed. To clarify the actual contents of C, NNH and S 8 in S 8 @CB@NNH hybrids, the powder samples thus undergo an acid immersion treatment followed by a thermogravimetric (TG) measurement (see experimental details in Methods section). The stepwise weight losses recorded in Fig. 2j reflect the detailed compositions of S 8 @CB@NNH, containing ∼ 8.2% of NNH, ∼ 13.4% of CB and ∼ 78.4% of active S 8 . Figure 2k shows the X-ray powder diffraction (XRD) pattern of S 8 @CB@NNH. In addition to distinguishable signals from NNH and amorphous CB, all other strong diffraction peaks stem from the crystalline S 8 (JCPDS no. 08-0247). Figure 2: Characterizations of the S 8 @CB@NNH bulky hybrids. ( a – d ) S.e.m. images of S 8 @CB@NNH hybrids. ( e – h ) EDX elemental mapping records towards one typical S 8 @CB@NNH bulky sample, and ( i ) a line-scan analysis on a selected section of this hybrid product. ( j ) A plot recording weight losses of S 8 @CB@NNH products during an acid immersion treatment combined with a TG measurement. ( k ) XRD pattern of synthesized S 8 @CB@NNH powders. Scale bars, 10 μm ( a , d ), 1 μm ( b ) and 100 nm ( c ). Full size image Electrochemical performance To evaluate the electrochemical properties of S 8 @CB@NNH hybrids, the as-synthesized electrodes are initially subjected to a long-term cyclic test in a potential window of ∼ 1.5–3 V at a constant current rate of 0.2 C (335 mA g −1 ; 1C=1,672 mA g −1 ). To verify and highlight the cooperative functions of NNH, bare S 8 @CB cathodes are also measured underneath the same conditions for comparison ( Fig. 3a ). The S 8 @CB cathode, as a whole, exhibits poor electrochemical behaviours including rapid decay in both specific capacity and coulombic efficiency and short cyclic life period. The discharge capacity on the first cycle achieves 1,345 mAh g −1 but it declines ceaselessly to a low capacitive value (less than ∼ 200 mAh g −1 after 300 cycles). On cycling, an increasing divergence between the charge and discharge capacity highly suggests the severe degradation on the coulombic efficiency. At the 300th cycle, only a coulombic efficiency value of ∼ 52% is sustained. The drastic decrease in capacity/coulombic efficiency would be mainly attributed to formidable kinetic issues in Li/S cell systems. A fraction of yielded polysulfide molecules that should be trapped in carbon reservoirs gradually migrate out of the cathode, and they may not be reversibly used again [32] . Even worse, undesired side reactions between these highly reactive polysulfide anions and electrolyte solvents would furthermore speed up the capacity losses [33] . By sharp contrast, the S 8 @CB@NNH cathode shows far better charge/discharge performance over 500 cycles. Among initial few cycles, the capacity of S 8 @CB@NNH in the beginning drops from the initial ∼ 968 mAh g −1 to a bottom level of ∼ 786 mAh g −1 (ninth cycle), which is mostly due to a delayed electrolyte infiltration into a well-capsulated structure. In subsequent 100 cycles (from the 50th to 150th cycle), the output for S 8 @CB@NNH-based cells rises progressively (since more S 8 becomes activated) until an electrochemical equilibrium state is built. About 150 cycles later, the capacity grows slowly to a maximum reversible value of ∼ 1,326 mAh g −1 (410th cycle) and maintains stabilized at ∼ 1,250 mAh g −1 to the end of cycling (no similar capacity-rise phenomena happen on S 8 @CB cathodes). Capacitive growth in this stage may be attributed to unavoidable structural fatigue/damage of outer layers because film breaking may provide new open-up places and accordingly more available routes for Li + to reach inner deep regions wherein the S 8 is deadly trapped. Till the 300th cycle, the S 8 @CB@NNH cathode still stably outputs a capacity of ∼ 1,164 mAh g −1 , almost six times greater than that of S 8 @CB. Also notice that unlike S 8 @CB-based cells, there is actually no capacity fading for S 8 @CB@NNH cathodes within prime 410 cycles. The coulombic efficiency always stays beyond ∼ 98%, indicative of outstanding electrochemical reversibility of S 8 @CB@NNH cathodes. Assuming the utilized S 8 is fully activated and contributes a theoretical capacity, the utilization ratio of active S 8 (calculated based on the maximum capacity in cycling) reaches up to ∼ 78.3%, with a substantial rise by 59.5% in contrast with that in S 8 @CB case (49.1%). Above evidences fully confirm that our facile encapsulation of NNH indeed plays a positive role in inhibiting the outward diffusion of long-chain soluble polysulfides from the cathode, and thus greatly promoting the long-cyclic cell performance. 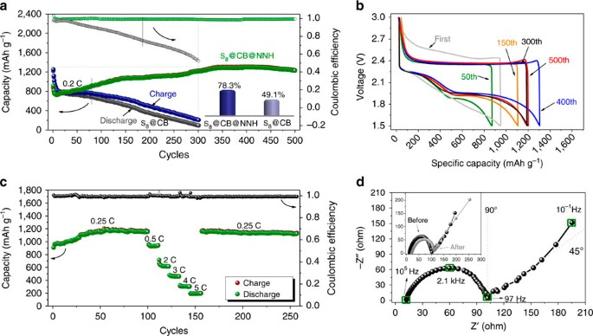Figure 3: Cell performance of the S8@CB@NNH hybrids. (a) Long-term cyclic testing of S8@CB@NNH and S8@CB at a current rate of 0.2 C in a potential window of∼1.5–3 V. The inset shows their utilization ratio of active S8. (b) Charge/discharge voltage profiles, (c) programmed cyclic responses and (d) electrochemical impedance spectrum of S8@CB@NNH cathode. Figure 3: Cell performance of the S 8 @CB@NNH hybrids. ( a ) Long-term cyclic testing of S 8 @CB@NNH and S 8 @CB at a current rate of 0.2 C in a potential window of ∼ 1.5–3 V. The inset shows their utilization ratio of active S 8 . ( b ) Charge/discharge voltage profiles, ( c ) programmed cyclic responses and ( d ) electrochemical impedance spectrum of S 8 @CB@NNH cathode. Full size image With the goal of attaining valuable insights into the cyclic information, we carefully analyze the charge/discharge voltage profiles of S 8 @CB@NNH cathode. For better comparisons between the pristine S 8 @CB and final S 8 @CB@NNH hybrid on cell performances, additional charge/discharge profiles of S 8 @CB have also been provided ( Supplementary Fig. 7 ). Figure 3b evidently shows that in the first electrochemical process, only a distorted discharge curve (rather than the smooth and distinct plateaus of bare S 8 @CB) is recorded. However, the discharge profiles lying at the 50th and subsequent cycles change a lot. Two main plateaus are present obviously, corresponding to the reduction of S 8 into complex solubilized polysulfides (for example, Li 2 S 8 , Li 2 S 6 , Li 2 S 4 and so on) over a potential range of ∼ 2.1–2.3 V and ultimate formation of solid-state Li 2 S 2 /Li 2 S at ∼ 2.0 V. Plateaus in later charge profiles are related to converse reactions from lithium sulfides to metastable polysulfides, and finally backward to the primitive S 8 . The appealing capacity-rise phenomenon is also recognized. The discharge plateau nearby ∼ 2.0 V extended gradually along with increased cyclic numbers, signifies that certain enhanced capacities are tightly correlated with complex conversions between highly ordered polysulfides and short-chain Li 2 S 2 /Li 2 S. We consider that the inner deep dispersions of active S 8 and postponed electrolyte penetration led by outer enclosure of NNH multi-layers may well account for the presence of this unique capacitive activation. Apart from that, frequent Li + migrations would endow exterior NNH layers with tiny micropore/mesopore architectures, quite favourable for Li + diffusion; as a consequence, better utilization of S 8 actives and easier conversion reactions of Li 2 S 4 /Li 2 S can be observed due to progressively enhanced electrochemical kinetics. Rate capabilities are further estimated by a cyclic test under programmed current densities ( Fig. 3c ). Corresponding charge/discharge voltage profiles at varied current rates are also displayed in Supplementary Fig. 8 . The cell exhibits a stable cyclic behaviour at each current speed, with all coulombic efficiencies nearly approaching ∼ 100%. Allowing for sufficient electrode activation, the S 8 @CB@NNH cathode preliminarily suffers from continuous 100 cycles under a constant current rate of 0.25 C, with a delivered capacity of ∼ 1,153 mAh g −1 (at the 100th cycle). Afterwards, the cell runs sequentially at 0.5, 2, 3, 4 and 5 C, enabling an output discharge capacity of ∼ 943, ∼ 610, ∼ 467, ∼ 289 and ∼ 195 mAh g −1 , respectively. This electrode rate performance is much superior to those in previous examples having similar ‘S 8 -in-carbon matrix’ configurations [34] , [35] , [36] . Even when the current rate suddenly switches back to 0.25 C, an exceptional specific capacity of 1,149 mAh g −1 is able to be retained (almost ∼ 100% recovery ratio in stored capacity). Figure 3d presents the electrochemical impedance spectrum of assembled S 8 @CB@NNH cells at an open-circuit voltage. The hybrid electrode of S 8 @CB@NNH, albeit with an exterior package of NNH films, shows a comparable semicircle diameter to bare S 8 @CB cathodes among the high-frequency region ( Supplementary Fig. 9 ). There are no considerable differences in terms of charge-transfer resistance ( R ct ), representing that such incorporation of NNH thin layers would not have a great effect on charge transfer. Moreover, little change is observed on R ct impedance (see the inset in Fig. 3d ) between original cells and the ones after 400 fatigue cycles, once again ensuring the good electrochemical stability of S 8 @CB@NNH cathode. Working principles of NNH for prolonged Li/S cells To make certain the change on discharge voltage profiles aforementioned, a cyclic voltammetry (CV) test at a slow scan rate of 50 μV s −1 is conducted ( Fig. 4a ). Besides reduction peaks that relates to the transformation of Li polysulfides to Li 2 S x , there seems other broad current responses emerging when cells are first scanned from 3.0 to 1.5 V. This unusual phenomenon may be greatly associated with undesired electrode polarizations/potential sluggish due to the presence of NNH outer films that would retard the electrolyte penetration and Li + transfer. In subsequent second and fourth cathodic scans, the intensity of these current signals is gradually diminished. Whereas, in the 10th scan, two well-defined reduction peaks above ∼ 2.0 V are present, and very little current trace in a potential scope of ∼ 1.64–1.8 V is noticed. We suppose that these current signals appearing in the low potential range (<1.85 V) should be linked to electrochemical interactions among the electrolyte, Li + and NNH. To prove this consumption, a CV scan towards the CB@NNH hybrids (without active S 8 ) under the same electrochemical conditions is performed ( Fig. 4b ). In the initial CV scan, there emerges a strong irreversible current peak (its intensity is still negligible when compared with that for S 8 -contained cases) located at the position of ∼ 1.5–1.86 V whose potential scope is highly in line with our records in Fig. 4a . This result may properly support our above estimation. With the increase of CV scans, the intensity for such current signals tends to decrease gradually and at last almost vanishes over 10 cycles, which implies the termination of these irreversible reactions. This electrochemical process may lead to the vast generation of complex Li, Ni-mixed hydroxides on S 8 @CB particle surface. 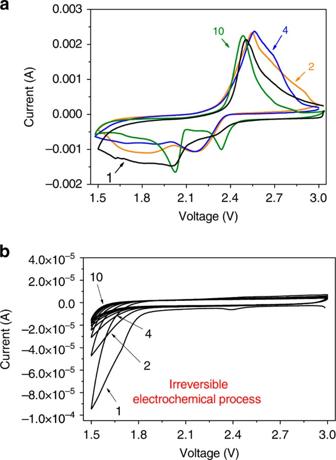Figure 4: Electrochemical characterizations of the S8@CB@NNH cathode. CV testing of (a) S8@CB@NNH cathode and (b) CB@NNH under a scan rate of 50 μV s−1. Figure 4: Electrochemical characterizations of the S 8 @CB@NNH cathode. CV testing of ( a ) S 8 @CB@NNH cathode and ( b ) CB@NNH under a scan rate of 50 μV s −1 . Full size image Deep understanding on the working principles of NNH in Li/S cells is made using ex situ s.e.m. monitoring coupled with precise EDX probing, Raman spectroscopy, XRD and surface-sensitive X-ray photoelectron spectroscopy (XPS) measurements based on the disassembly of cycled cells at the charge-end state of 50th, 300th and 500th, respectively. 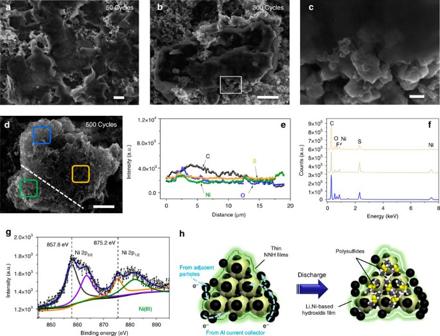Figure 5: Characterizations of cycled S8@CB@NNH cathodes. (a–d) Theex situs.e.m. monitoring the cathodic morphological changes on increased cyclic numbers. EDX probing towards the S8@CB@NNH cathode after 500 cycles: (e) a line-scan analysis and (f) EDX records on different particle zones. (g) High-resolution Ni 2p XPS spectrum and (h) a schematic showing working mechanisms of NNH in Li/S cathodes. Proper pathways for electron transfer in the discharge stage have also been displayed. Scale bars, 10 μm (a,b,d) and 100 nm (c). Figure 5a–d in turn displays representative s.e.m. images of disassembled cells after different cycles. The top-view s.e.m. image ( Fig. 5a ) clearly depicts that bulky S 8 @CB@NNH particles remain densely packed and well embedded in the film electrode after 50 times of full charge. In addition, there are layered structures definitely filled in electrode matrices. The electrode suffering from 300 continual cycles looks similar to that in the former case. Though the cathode film to some extent becomes loose possibly due to volume expansions and structural reconfigurations of electrode during lithiation/delithiation, the close encapsulation of protective armors on S 8 @CB particles is always maintained ( Fig. 5b ). Attentions to morphological features of cycled S 8 @CB@NNH have been paid specially. A zoom-in s.e.m. observation on a selected edge place ( Fig. 5c ) discloses that the subunits of S 8 @CB@NNH (size: 50 ∼ 150 nm, a bit larger than pristine S 8 @CB unit) are still underneath the protection of gel-like film structures despite the situation that cells have run uninterruptedly for hundreds of cycles. The geometric observation on the cathode ( Fig. 5d ) unambiguously demonstrates that bulks of S 8 @CB@NNH, though turning into porous structures in whole or in part, are able to survive a long-time cyclic test over 500 times charge and discharge (lasting for more than half a year) and still preserve an integrated electrode construction. Line-scan analysis across one cycled S 8 @CB@NNH particle ( Fig. 5e ) exhibits a uniform elemental distribution of C, S, O and Ni, proving that the functionalized hybrid configurations cannot be varied tremendously even if suffering from long-term input/output operations. EDX testing towards different particle zones ( Fig. 5f ) give out an identical result, reconfirming the good retention ability on electrode constituents. XRD measurement is used to identify the chemical compositions of cycled S 8 @CB@NNH after 50 cycles ( Supplementary Fig. 10a ). The presence of a broad diffraction signal instead of original sharp peaks illustrates that the primal S 8 crystals have evolved into an amorphous state. Moreover, a wide (001) diffraction peak also turns up at 20.4 o , which is well indexed to the (001) phase of LiOH (JCPDS no. 32-0564). To illustrate LiOH comes from reactions between Li + and NNH, Raman spectroscopy is implemented on cycled electrode of CB@NNH purposely. In Raman spectrum ( Supplementary Fig. 10b ), we readily distinguish the characteristic peaks of LiOH, which are successively assigned to A 1g mode (329 cm −1 ) and E g mode (531 cm −1 and 620 cm −1 ) [37] , revealing a fact that LiOH is indeed produced after irreversible electrochemical reactions mentioned above. XPS testing is further used to determine the chemical state of Ni in the formed composites coating on S 8 @CB. High-resolution Ni 2p XPS spectrum ( Fig. 5g ) shows that two prominent peaks (indexed to Ni 2p 3/2 and Ni 2p 1/2 ) are located at binding energies of 857.8 and 875.2 eV, with satellite peaks at high binding energies of 863.5 and 880.4 eV, respectively. All these features have been fully evidenced in the literatures as typical fingerprints of Ni(III) oxidation state (rather than the initial Ni(II) state) [38] . The variation in chemical valence hints that the involved Ni element in armors may also take part in redox reactions, possibly acting as a mediator/catalyst role via interactions with polysulfides to improve the reaction kinetics [40] , and contribute to the cell capacity (thus the total specific capacity is even a bit higher than that of S 8 ). To further understand the interactions among pure NNH (exclude CB since CB itself has a reversible capacity when working in cell systems), Li + and polysulfides in Li/S cells, more systematic researches will be highly encouraged and concentrated in our future work via using distinct binders (like CMC, LA132 and so on). The CV comparisons between the S 8 @CB@NNH and S 8 @CB electrodes after 100 cycles ( Supplementary Fig. 11 ) may grant us important hints to account for the capacity exceeding as well as extended plateaus. Clearly, S 8 @CB@NNH exhibits a higher current intensity than S 8 @CB owing to its preferable capacity retention. Notice that except for signal increases at/around peak positions, additional current enhancements are found in other potential regions (for example, from ∼ 2.0 to 2.3 V) as well. This implies that besides electrochemical reactions of S 8 (the main capacity contributor), other gentle reversible conversions in cathode systems (typically like pseudocapacitive and inner redox reactions or interactions and so on) may give partial contributions to the ultimate cell capacity. Figure 5: Characterizations of cycled S 8 @CB@NNH cathodes. ( a – d ) The ex situ s.e.m. monitoring the cathodic morphological changes on increased cyclic numbers. EDX probing towards the S 8 @CB@NNH cathode after 500 cycles: ( e ) a line-scan analysis and ( f ) EDX records on different particle zones. ( g ) High-resolution Ni 2p XPS spectrum and ( h ) a schematic showing working mechanisms of NNH in Li/S cathodes. Proper pathways for electron transfer in the discharge stage have also been displayed. Scale bars, 10 μm ( a , b , d ) and 100 nm ( c ). Full size image Above characteristics and evidences guide us to unveil the working mechanism of NNH in Li/S cathodes, as schematically described in Fig. 5h . Among primal tens of cycles, the majority of thin-layered NNHs surrounding the S 8 @CB particles are gradually transformed into more electrochemically stabilized Li-based hydroxide compounds via mild irreversible discharge reactions without causing any structure collapses or film pulverizations. Abundant incorporation of hydrophilic and surface hydroxyl groups that are reported to bind favourably with polysulfide anions [12] , [39] , combined by a good physicochemical stability of such derived substances could effectively assure the suppression of polysulfides dissolution and leakage. This has been testified by good electrochemical properties of S 8 @CB@NNH, with remarkable extended cyclability, greatly enhanced S 8 utilization and fairly high coulombic efficiencies (all the time retaining ∼ 98% above). Moreover, the multi-layered armors compactly ‘worn’ on S 8 @CB would never deteriorate the ionic transfer property. On one hand, rich Li + in electrolyte phase may enter the inner places of S 8 @CB@NNH by means of Li + exchange with Li, Ni-mixed hydroxides wrapping outside the S 8 @CB. On the other hand, the massive and rapid ionic migrations/diffusions can proceed smoothly throughout effortlessly traversing micropores/mesopores that intrinsically exist on NNH films or in situ created by Li + on thin-layered structures during deep charge/discharge cycling. In this work, the thin-layered Ni-based hydroxide has been demonstrated for the first time as one feasible and effective encapsulation material to prolong the service life of Li/S cells. Our uncustomary selection of hydroxides as an encapsulation candidate is highly triggered by three critical factors as follows: First and foremost, there exist electrochemically irreversible interactions between Li + and layered hydroxides, leading to the generation of a more stabilized shelly structure. This shelly structure can function as a robust protective layer to entrap the active S 8 and intermediate polysulfide molecules inside the cathodes, hence efficiently extending the cell cycle lifespan. Next, our used layered NNH itself is pretty thin. With that, this gauzy covering layer allows the ease of Li + access into the cathode either by diffusions across both interspaces and micropores/mesopores or via Li + exchanges occurring on the solid–liquid interface. This ionic transit is much easier than other cases for thick physical barriers. Last but never the least, the thin, soft and flexible film prepared in solution phase is apt to worn uniformly on involved precursors no matter what forms and shapes they are present in. This general and simple synthetic strategy, thereby, would pledge the mass production of integrated core–shell hybrid constructions with both intact and intimate wrapping properties. As a proof-of-concept demonstration, our designed S 8 @CB@NNH hybrid cathode proves great improvements in capacity retention and long-cyclic ability. Unlike previous approaches to trap polysulfides by physical barriers or simple surface interactions, our method is quite efficient, simple, cost-effective and particularly suitable for bulky materials, opening up the prospect of using layered thin-metal hydroxides as a creative and effective class of encapsulation materials for promotions of Li/S cell performance. Despite these advances, in the way still stand formidable challenges, typically like the presence of undesired potential sluggish/polarizations associated with increased charge-transfer resistances due to tight capsulations of NNH. To decrease such polarizations during the cell operation, further development of better thin shells/layers by means of proper and smart engineering/hybridization of NNH with other robust and conductive substances may hold great promise in future Li/S cell technology and deserve our systematic and elaborate studies. Preparation of S 8 @CB hybrid The S 8 @CB hybrid was prepared following a melt-diffusion strategy. S 8 powders (8 g; Sigma-Aldrich, Index-No. 016-094-00-1; assay ≥99.5%) and CB (2 g; LITX 50, Cabot China (Shanghai) Ltd.; ∼ 45–60 m 2 g −1 ) were grounded together (the optimal weight ratio of S 8 /CB was found to be 4:1), and then heated to 155 °C and maintained for 6 h. Preparation of S 8 @CB@NNH hybrid The S 8 @CB@NNH hybrid was synthesized by using S 8 @CB hybrids as the starting materials. In details, a mixture of S 8 @CB powders (0.6 g), hexamethylenetetramine/C 6 H 12 N 4 , 0.5 g (Sigma-Aldrich, Index-No. 612-101-00-2; assay ≥99.0%), Ni(NO 3 ) 2 ·6H 2 O (0.25 g; Sigma-Aldrich, Index-No. 028-012-00-1; assay ≥97.0%) and distilled water (50 ml) was magnetically stirred for 30 min. Afterwards, the resulting suspension was transferred into a sealed container (80 ml) and held at 95 °C for 6 h. Samples were then collected, washed by distilled water several times and dried at 60 °C in electronic oven. Characterization The powder samples were characterized by field-emission SEM (JSM-6700F, 5.0 kV) collocated with a high-precision energy dispersive spectroscopy system (Oxford Instruments of X-Max N ; its silicon drift detector comes in a wide range of detecting sizes, from 20 mm 2 for microanalysis up to an astounding 150 mm 2 for advanced nanoanalysis), XRD (Bruker D8 Advance diffractometer with Cu Kα radiation, λ =0.15418, nm) and N 2 adsorption/desorption (ASAP2020 volumetric adsorption analyser; Micromeritics, USA). The morphology and crystalline structure of NNH were further characterized using a TEM/high-resolution TEM (JEM 2100F). XPS spectrum was measured on a Perkin-Elmer model PHI 5600 XPS system with a resolution of 0.3–0.5 eV from a monochromated aluminium anode X-ray source. Electrical properties were recorded by the use of a Keithley 4200 semiconductor characterization system (USA). The Raman spectrum was made by using a WITec CRM200 Raman system with 532 nm excitation laser. TG analysis was performed on a SDT600 apparatus under a heating rate of ∼ 5 K min −1 in Ar atmosphere. For the acid immersion treatment, 1 g of fresh S 8 @CB@NNH hybrid powder was put into a 100 ml glass beaker wherein a 60 ml of 3 M hydrochloric acid (HCl) solution was contained. This mixture was then subjected to a 30 min of mild magnetic stirring (rotating rate: 200 r min −1 ) so as to guarantee the complete removal of NNH. The next sample collection procedure is much crucial to the acid immersion treatment. Powders were carefully collected via a slow vacuum filtration process using a microporous membrane filter (Nylon 66; pore size: 0.22 μm), washed with deionized water several times and dried under vacuum conditions at room temperature. To avoid weight losses, nearly all of the residuals on container are thoroughly collected. The powder mass was then determined by a microbalance with an accuracy of 0.01 mg (A&D Company N92, Japan). According to mass differences, NNH statistically took up ∼ 8.2% in S 8 @CB@NNH hybrids. Electrochemical measurements The working electrodes were all prepared by mixing powder samples with polyvinylidene difluoride (Sigma-Aldrich, Product No. 427152) binder and CB (weight ratio: 80:10:10) in N -methyl-2-pyrrolidone (Sigma-Aldrich, assay ≥99%) to form a slurry, which was then pasted onto aluminium foil and dried in an electrical oven. Bare S 8 @CB and CB@NNH electrodes were also made in the same way for electrochemical comparisons. The 2032-type coin cells were then assembled in an Ar-filled glovebox (MBRAUN, UNIlab, Germany) by using Li foil as the counter electrode. The used electrolyte was lithium bis(trifluoromethanesulphonyl)imide (1 M) in 1:1 (v/v) 1,2-dimethoxyethane and 1,3-dioxolane (Fosai New Material Co., Ltd. and Kanagawa Co., Ltd., Japan). LiNO 3 salt was added (1 wt%) to help passivate the Li anode surface. The mass of electrode materials was measured on a high-accuracy microbalance. The mass ratio of S 8 in synthesized S 8 @CB@NNH hybrid is ∼ 78%, while the ratio value in pasted electrodes is ∼ 62.4% due to additives of CB and polyvinylidene difluoride. For one electrode, the typical mass loading was ∼ 1.8–2.5 mg cm −2 unless otherwise stated. The specific capacity values are calculated based on the total mass of electrode materials (excluding CB and polymer binders). In cell testing, the charge/discharge profiles and cyclability data were obtained with a programmable battery cycler (Neware Instruments). The C rates specified in this case study are based on the mass and theoretical capacity of S 8 (1C=1,675 mA g −1 ). All cells were aged for 8 h before the cyclic test. How to cite this article: Jiang, J. et al. Encapsulation of sulfur with thin-layered nickel-based hydroxides for long-cyclic lithium–sulfur cells. Nat. Commun. 6:8622 doi: 10.1038/ncomms9622 (2015).